Angiotensin inhibition enhances drug delivery and potentiates chemotherapy by decompressing tumour blood vessels Cancer and stromal cells actively exert physical forces (solid stress) to compress tumour blood vessels, thus reducing vascular perfusion. Tumour interstitial matrix also contributes to solid stress, with hyaluronan implicated as the primary matrix molecule responsible for vessel compression because of its swelling behaviour. Here we show, unexpectedly, that hyaluronan compresses vessels only in collagen-rich tumours, suggesting that collagen and hyaluronan together are critical targets for decompressing tumour vessels. We demonstrate that the angiotensin inhibitor losartan reduces stromal collagen and hyaluronan production, associated with decreased expression of profibrotic signals TGF-β1, CCN2 and ET-1, downstream of angiotensin-II-receptor-1 inhibition. Consequently, losartan reduces solid stress in tumours resulting in increased vascular perfusion. Through this physical mechanism, losartan improves drug and oxygen delivery to tumours, thereby potentiating chemotherapy and reducing hypoxia in breast and pancreatic cancer models. Thus, angiotensin inhibitors —inexpensive drugs with decades of safe use — could be rapidly repurposed as cancer therapeutics. Drug and oxygen delivery in tumours is dependent on the organization and efficiency of perfused vessels [1] , [2] , [3] . Solid stress (pressure from solid tissue components) accumulates in tumours as cancer and stromal cells proliferate in a confined microenvironment created by crosslinked matrix molecules [4] , [5] , [6] . The matrix stores and transmits this stress throughout the tumour [7] , collapsing blood vessels to limit perfusion [8] , [9] . Meanwhile, patients with low tumour perfusion—presumably with extensive hypoxia and impaired drug delivery—show poorer chemotherapy responses and shorter survival versus patients with high perfusion [10] , [11] . Thus, there is an urgent need for drugs that can target solid stress to improve blood perfusion and drug delivery in tumours. Stromal cells and matrix contribute to solid stress, but the mechanisms through which these components interact to compress tumour vessels remain unclear. Uncovering these mechanisms could lead to novel paradigms for enhancing tumour perfusion. In this study, we show that different tumour matrix components produced by cancer-associated fibroblasts (CAFs) collaborate to compress vessels. We demonstrate that angiotensin signalling blockade inactivates CAFs to reduce their production of these matrix components while also reducing CAF density. Through this mechanism, we find that angiotensin receptor blockers (ARBs) reduce solid stress, decompress tumour vessels, increase drug and oxygen delivery and improve chemotherapy outcomes. Thus, solid stress can be targeted by decreasing CAF activity and agents that do so can improve tumour perfusion and enhance chemotherapy. Hyaluronan and collagen collaborate to compress tumour blood vessels Hyaluronan has been proposed to be the primary matrix molecule responsible for vessel compression [12] , but its exact mechanism remains unclear. Hyaluronan interacts with collagen in a complex manner [13] , and both contribute to the accumulation of solid stress through these interactions [5] . Thus, we examined whether collagen may also affect vessel compression ( Fig. 1a,b ). We measured vessel perfusion (patency) in multiple orthotopic tumours and compared it with hyaluronan and collagen levels. Interestingly, we found that both hyaluronan and collagen area fraction were inversely associated with perfused vessel fractions ( Fig. 1c ). The mean of these matrix area fractions had an even stronger inverse correlation with perfusion, indicating a complex nonlinear relationship between the two matrix molecules and perfusion. Surprisingly, we found that vessel perfusion did not correlate with hyaluronan area fractions in tumours with low collagen levels ( Fig. 1d ); rather, hyaluronan and perfusion were inversely correlated only in collagen-rich tumours. In contrast, perfusion inversely correlated with collagen area fraction in both hyaluronan-rich and hyaluronan-poor tumours ( Fig. 1e ). These findings indicate that collagen is needed for hyaluronan to exert compression on blood vessels, suggesting that both are potential targets for vessel decompression in desmoplastic tumours. 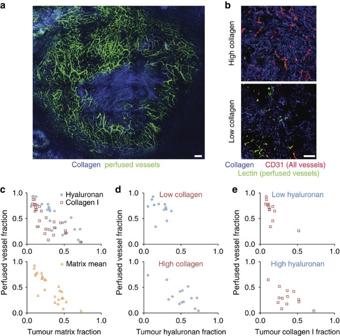Figure 1: Collagen and hyaluronan interact to compress tumour blood vessels. (a) Representative image from intravital multiphoton microscopy of perfused tumour vessels (green) and collagen (blue), showing that high collagen levels colocalize with low perfusion in an E0771 breast tumour. Scale bar, 200 μm. (b) Histology images of vascular perfusion in orthotopic AK4.4 pancreatic tumours with high versus low collagen levels. High local collagen I levels (blue) appear to colocalize with collapsed vessels (red, collapsed; green/yellow, perfused)in vivo. Scale bar, 100 μm. (c) Correlation of perfused vessel fraction versus tumour matrix area fractions in multiple orthotopic pancreatic tumour models (AK4.4 and L3.6pl) in mice. Following lectin injection and animal killing, perfusion was quantified as the fraction of vessels that are both lectin- and CD31-positive out of all CD31-positive vessels. Perfusion inversely correlates with both hyaluronan (R=−0.79,P<0.001, Pearson’s correlation) and collagen I (R=−0.78,P<0.001, Pearson’s correlation), but has a stronger inverse correlation (R=−0.86,P<0.001, Pearson’s correlation) with the average matrix area fraction. (d) Grouping these tumours into those with either low (<17%) or high (≥17%) collagen reveals that perfusion does not correlate (R=−0.33, Pearson’s correlation) with hyaluronan in collagen-poor tumours but does inversely correlate (R=−0.71,P=0.004, Pearson’s correlation) in collagen-rich tumours. (e) In contrast, grouping the tumours into those with either low (<33%) or high (≥33%) hyaluronan shows that perfusion inversely correlates with collagen I in both hyaluronan-poor (R=−0.73,P=0.003, Pearson’s correlation) and hyaluronan-rich (R=−0.57,P=0.040, Pearson’s correlation) tumours. Figure 1: Collagen and hyaluronan interact to compress tumour blood vessels. ( a ) Representative image from intravital multiphoton microscopy of perfused tumour vessels (green) and collagen (blue), showing that high collagen levels colocalize with low perfusion in an E0771 breast tumour. Scale bar, 200 μm. ( b ) Histology images of vascular perfusion in orthotopic AK4.4 pancreatic tumours with high versus low collagen levels. High local collagen I levels (blue) appear to colocalize with collapsed vessels (red, collapsed; green/yellow, perfused) in vivo . Scale bar, 100 μm. ( c ) Correlation of perfused vessel fraction versus tumour matrix area fractions in multiple orthotopic pancreatic tumour models (AK4.4 and L3.6pl) in mice. Following lectin injection and animal killing, perfusion was quantified as the fraction of vessels that are both lectin- and CD31-positive out of all CD31-positive vessels. Perfusion inversely correlates with both hyaluronan ( R =−0.79, P< 0.001, Pearson’s correlation) and collagen I ( R =−0.78, P <0.001, Pearson’s correlation), but has a stronger inverse correlation ( R =−0.86, P <0.001, Pearson’s correlation) with the average matrix area fraction. ( d ) Grouping these tumours into those with either low (<17%) or high (≥17%) collagen reveals that perfusion does not correlate ( R =−0.33, Pearson’s correlation) with hyaluronan in collagen-poor tumours but does inversely correlate ( R =−0.71, P =0.004, Pearson’s correlation) in collagen-rich tumours. ( e ) In contrast, grouping the tumours into those with either low (<33%) or high (≥33%) hyaluronan shows that perfusion inversely correlates with collagen I in both hyaluronan-poor ( R =−0.73, P =0.003, Pearson’s correlation) and hyaluronan-rich ( R =−0.57, P =0.040, Pearson’s correlation) tumours. Full size image Angiotensin inhibition reduces stromal fibrosis signalling We therefore sought a translatable therapy that targets both collagen and hyaluronan. We recently found that the ARB losartan can reduce collagen I production in CAFs by downstream inhibition of transforming growth factor (TGF)-β1 activation [14] , [15] through thrombospondin-1 (TSP-1) inhibition [16] , [17] , [18] . As hyaluronan synthesis is similarly TGF-β1 dependent, we expected that losartan would also decrease hyaluronan production. We generated transgenic FVB mice expressing the fluorescent protein dsRed driven by the promoter for α-smooth-muscle actin (αSMA) [19] , a marker for activated CAFs. In these mice ( αSMA P -dsRed/FVB ), we orthotopically implanted AK4.4 pancreatic tumour cells, treated these mice with losartan or saline (control), and then isolated the CAFs (activated pancreatic stellate cells) from their tumours using fluorescence-activated cell sorting ( Supplementary Fig. S1 ). We confirmed that CAF expression of TGF-β1 and collagen I was reduced by losartan ( Fig. 2a,b ). We then measured expression of hyaluronan synthases 1–3 in these CAFs and found that hyaluronan synthases 1–3 were also greatly decreased by losartan ( Fig. 2a,b ). Thus, losartan is a dual inhibitor of stromal collagen and hyaluronan production. 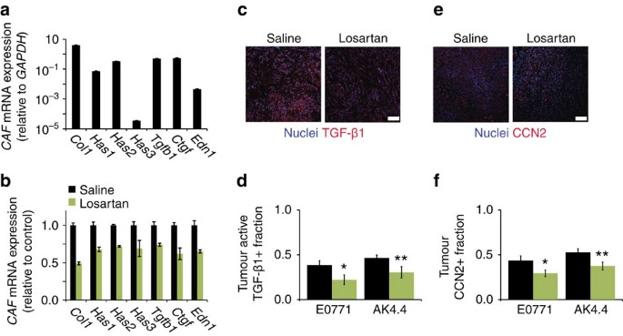Figure 2: Losartan decreases profibrotic stromal activity in tumours. (a) Expression levels of fibrosis-related genes in murine cancer-associated fibroblasts (CAFs) isolated from orthotopic AK4.4 pancreatic tumours. AK4.4 tumours were orthotopically implanted inαSMAP-dsRed/FVBmice, resulting in αSMA+ CAFs that express dsRed. These mice were treated with losartan or saline (control), then the CAFs from their tumours were isolated using fluorescence-activated cell sorting for dsRed. The isolated control CAFs express high mRNA levels of collagen I (Col1), hyaluronan synthases (HAS)1–2 (Has1,Has2), TGF-β1 (Tgfb1) and CCN2 (Ctgf), with low levels of HAS 3 (Has3) and moderate levels of ET-1 (Edn1). Levels normalized to GAPDH expression. (b) Comparison of expression levels of fibrosis-related genes in the CAFs isolated from losartan- or saline-treated (control) mice. Losartan reduces the mRNA expression of each of these profibrotic genes in CAFs (P<0.05, Student’st-test). Levels normalized to saline control. (c) Histology images showing the effect of losartan on tumour TGF-β1 expression. Scale bar, 100 μm. (d) Immunohistochemical analysis of TGF-β1 expression with losartan treatment. Losartan reduces the expression of TGF-β1 in E0771 (*P=0.048, Student’st-test) and AK4.4 tumours (**P=0.044, Student’st-test). (e) Histology images showing the effect of losartan on tumour CCN2 expression. Scale bar, 100 μm. (f) Immunohistochemical analysis of CCN2 expression with losartan treatment. Losartan reduces the expression of CCN2 in E0771 (*P=0.044, Student’st-test) and AK4.4 (**P=0.046, Student’st-test) tumours. Scale bar, 100 μm. Animal numbersn=4 (CAF expression),n=7–8 (E0771 TGF-β1, CCN2),n=4–6 (AK4.4 TGF-β1, CCN2). Error bars indicate s.e.m. Figure 2: Losartan decreases profibrotic stromal activity in tumours. ( a ) Expression levels of fibrosis-related genes in murine cancer-associated fibroblasts (CAFs) isolated from orthotopic AK4.4 pancreatic tumours. AK4.4 tumours were orthotopically implanted in αSMA P -dsRed/FVB mice, resulting in αSMA+ CAFs that express dsRed. These mice were treated with losartan or saline (control), then the CAFs from their tumours were isolated using fluorescence-activated cell sorting for dsRed. The isolated control CAFs express high mRNA levels of collagen I ( Col1 ), hyaluronan synthases (HAS)1–2 ( Has1 , Has2 ), TGF-β1 ( Tgfb1 ) and CCN2 ( Ctgf ), with low levels of HAS 3 ( Has3 ) and moderate levels of ET-1 ( Edn1 ). Levels normalized to GAPDH expression. ( b ) Comparison of expression levels of fibrosis-related genes in the CAFs isolated from losartan- or saline-treated (control) mice. Losartan reduces the mRNA expression of each of these profibrotic genes in CAFs ( P <0.05, Student’s t -test). Levels normalized to saline control. ( c ) Histology images showing the effect of losartan on tumour TGF-β1 expression. Scale bar, 100 μm. ( d ) Immunohistochemical analysis of TGF-β1 expression with losartan treatment. Losartan reduces the expression of TGF-β1 in E0771 (* P= 0.048, Student’s t -test) and AK4.4 tumours (** P= 0.044, Student’s t -test). ( e ) Histology images showing the effect of losartan on tumour CCN2 expression. Scale bar, 100 μm. ( f ) Immunohistochemical analysis of CCN2 expression with losartan treatment. Losartan reduces the expression of CCN2 in E0771 (* P= 0.044, Student’s t -test) and AK4.4 (** P= 0.046, Student’s t -test) tumours. Scale bar, 100 μm. Animal numbers n =4 (CAF expression), n =7–8 (E0771 TGF-β1, CCN2), n =4–6 (AK4.4 TGF-β1, CCN2). Error bars indicate s.e.m. Full size image Losartan rapidly reduces established tumour matrix levels [14] , which implies that it degrades or destabilizes matrix through an uncharacterized mechanism in addition to preventing matrix production through TGF-β1. Connective tissue growth factor (CCN2/CTGF), a matricellular protein, stabilizes the transient fibrosis produced by TGF-β1 activity [20] , [21] and is downstream of angiotensin signalling through TGF-β1 in other fibrosis diseases [22] , [23] , suggesting that losartan could be destabilizing the matrix by inhibiting CCN2 expression. By comparing CAFs isolated from losartan- versus saline-treated mice, we found that losartan reduced expression of CCN2 ( Fig. 2a,b ). We next used immunohistochemistry to assess how losartan affects CCN2, active TGF-β1 and matrix levels in orthotopic E0771 and AK4.4 models, which recapitulate the desmoplasia observed in human mammary adenocarcinoma and in human pancreatic ductal adenocarcinoma, respectively ( Supplementary Figs S2–S4 ). Losartan reduced both CCN2 and active TGF-β1 in E0771 breast and AK4.4 pancreatic tumours ( Fig. 2c–f and Supplementary Fig. S5 ). Further, losartan decreased collagen I and hyaluronan in both of these tumours ( Fig. 3a–d and Supplementary Figs S4, S6 and S7 ). Thus, losartan decreases stromal matrix production through TGF-β1 while potentially destabilizing the existing matrix through CCN2. Collectively, these effects lead to a reduction in collagen and hyaluronan levels in desmoplastic tumours. 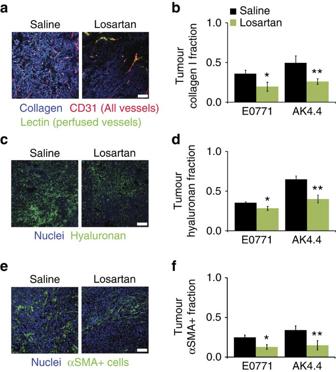Figure 3: Losartan reduces matrix and stromal density in tumours. (a) Histology images showing the effect of losartan on tumour collagen levels and perfusion. Scale bar, 100 μm. (b) Immunohistochemical analysis of tumour collagen levels following losartan treatment. Losartan decreases the collagen I-positive area fraction in E0771 (*P=0.040, Student’st-test) and AK4.4 (**P=0.022, Student’st-test) tumours. (c) Histology images showing the effect of losartan on tumour hyaluronan levels. Scale bar, 100 μm. (d) Immunohistochemical analysis of tumour hyaluronan levels following losartan treatment. Losartan also reduces the hyaluronan-positive area fraction in E0771 (*P=0.048, Student’st-test) and AK4.4 (**P=0.019, Student’st-test) tumours, as assessed using a hyaluronan-binding protein probe. (e) Histology images showing the effect of losartan on tumour αSMA+ CAF levels. Scale bar, 100 μm. (f) Immunohistochemical analysis of αSMA+ CAF density with losartan treatment. Losartan reduces the CAF density in E0771 (*P=0.019, Student’st-test) and AK4.4 (**P=0.040, Student’st-test) tumours. Animal numbersn=5–7 (E0771 collagen),n=4–6 (AK4.4 collagen),n=4–5 (E0771 hyaluronan),n=4 (AK4.4 hyaluronan),n=5 (E0771 αSMA),n=5–6 (AK4.4 αSMA). Error bars indicate s.e.m. Figure 3: Losartan reduces matrix and stromal density in tumours. ( a ) Histology images showing the effect of losartan on tumour collagen levels and perfusion. Scale bar, 100 μm. ( b ) Immunohistochemical analysis of tumour collagen levels following losartan treatment. Losartan decreases the collagen I-positive area fraction in E0771 (* P= 0.040, Student’s t -test) and AK4.4 (** P= 0.022, Student’s t -test) tumours. ( c ) Histology images showing the effect of losartan on tumour hyaluronan levels. Scale bar, 100 μm. ( d ) Immunohistochemical analysis of tumour hyaluronan levels following losartan treatment. Losartan also reduces the hyaluronan-positive area fraction in E0771 (* P= 0.048, Student’s t -test) and AK4.4 (** P= 0.019, Student’s t -test) tumours, as assessed using a hyaluronan-binding protein probe. ( e ) Histology images showing the effect of losartan on tumour αSMA+ CAF levels. Scale bar, 100 μm. ( f ) Immunohistochemical analysis of αSMA+ CAF density with losartan treatment. Losartan reduces the CAF density in E0771 (* P= 0.019, Student’s t -test) and AK4.4 (** P= 0.040, Student’s t -test) tumours. Animal numbers n =5–7 (E0771 collagen), n =4–6 (AK4.4 collagen), n =4–5 (E0771 hyaluronan), n =4 (AK4.4 hyaluronan), n =5 (E0771 αSMA), n =5–6 (AK4.4 αSMA). Error bars indicate s.e.m. Full size image Angiotensin inhibition decreases CAF density in tumours As the effects of losartan on matrix expression in tumours were pronounced, and as angiotensin signalling has been previously shown to activate fibroblasts in other fibrosis diseases [24] , [25] , we next tested whether losartan could also reduce CAF density. We found that losartan lowered the density of αSMA+ cells in E0771 and AK4.4 tumours ( Fig. 3e,f and Supplementary Fig. S8 ), indicating a decrease in activated CAFs. In other fibrotic diseases, fibroblast activation occurs through endothelin-1 (ET-1) expression [26] downstream of TGF-β1 [27] and angiotensin signalling [28] . Thus, we expected that losartan may reduce ET-1 expression by CAFs. Indeed, in the CAFs isolated from losartan- or saline-treated mice, we found that losartan decreased the expression of ET-1 ( Fig. 2a,b ). Therefore, losartan seems to reduce activation of fibroblasts or stellate cells to αSMA+ CAF phenotype, leading to a reduction in CAF density. AT1 and AT2 signalling opposingly affect tumour fibrosis To investigate how best to target angiotensin signalling, we next investigated the role of angiotensin receptor signalling in tumour desmoplasia. We first studied the effects of the angiotensin-converting enzyme inhibitor (ACE-I) lisinopril on the matrix, because ACE-Is block both angiotensin-II-receptor-1 (AT1) and angiotensin-II-receptor-2 (AT2) signalling. Intriguingly, lisinopril reduced collagen I and hyaluronan in AK4.4 tumours to a lesser extent than losartan, which blocks only AT1 signalling ( Supplementary Fig. S9 ). This suggests that AT2 inhibition leads to increased matrix levels in tumours, in opposition to AT1 inhibition. We confirmed this by implanting E0771 in knockout mouse models of AT1 ( Agtr1a −/− ) and AT2 ( Agtr2 −/− ). We found that tumours in the AT1-knockout mice had lower levels of collagen I and hyaluronan than tumours in wild-type mice ( Fig. 4a,b ), whereas the tumours in AT2-knockout mice had higher collagen I and hyaluronan levels than tumours in wild-type mice ( Fig. 4c,d ), indicating that stromal AT2 signalling inhibits tumour desmoplasia, whereas AT1 signalling promotes it. Importantly, this result fits with the known effects of angiotensin signalling on fibrosis in other diseases [29] , [30] , [31] . To confirm the relevance of stromal AT1 and AT2 inhibition, we measured the expression of these receptors in CAFs and cancer cells from wild-type mice. We found that CAFs isolated from AK4.4 tumours express far more AT1 and AT2 than AK4.4 or E0771 cancer cells ( Fig. 4e ). We confirmed this result with immunohistochemistry in E0771 tumours, where we found that a moderate fraction of CAFs in these tumours express AT1 at high levels, whereas most other cells express AT1 at low levels; most CAFs express high levels of AT2, whereas a small fraction of other cells express similar AT2 levels ( Fig. 4f,g ). These results indicated that the cellular targets of angiotensin blockers relating to matrix production are CAFs rather than cancer cells. Thus, the antidesmoplasia benefits of ARBs are because of specific AT1 inhibition in tumour stroma, and ACE-Is may not provide the same benefits due to combined AT1 and AT2 inhibition. 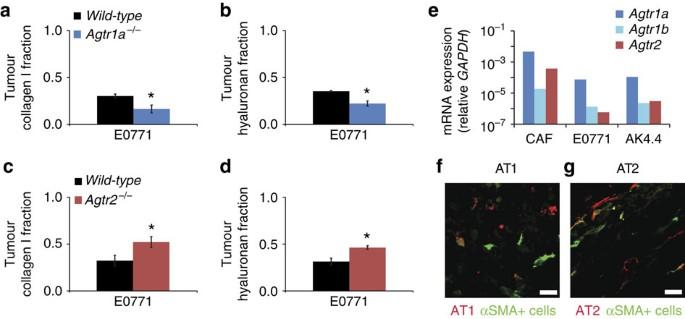Figure 4: Stromal angiotensin signalling induces matrix production in tumours. (a) Tumour collagen and (b) hyaluronan levels in angiotensin-II-receptor-1 (AT1)-knockout mice. Orthotopic E0771 breast tumours implanted in AT1-knockout mice (Agtr1a−/−) have (a) a lower collagen I area fraction (*P=0.026, Student’st-test) and (b) a lower hyaluronan area fraction (*P=0.011, Student’st-test) than E0771 tumours implanted in wild-type C57BL/6 mice. (c) Tumour collagen and (d) hyaluronan levels in angiotensin-II-receptor-2 (AT2) knockout mice. Orthotopic E0771 breast tumours implanted in AT2-knockout mice (Agtr2−/−) have (c) a higher collagen I area fraction (*P=0.047, Student’st-test) and (d) a higher hyaluronan area fraction (*P=0.012, Student’st-test) than E0771 tumours implanted in wild-type C57BL/6 mice. Tumours were time- and size-matched at ~200 mm3. (e) Expression of AT1 (Agtr1aandAgtr1bgenes) and AT2 (Agtr2gene) mRNA in murine cancer-associated fibroblasts (CAFs) and cancer cells. CAFs isolated from AK4.4 tumours express over one order of magnitude more AT1 than either E0771 or AK4.4 cancer cells. Similarly, the CAFs express over two orders of magnitude more AT2 than either E0771 or AK4.4 cells. (f) Expression of AT1 (red) in αSMA+ CAFs (green) and cancer cells in tumours. We imaged CAFs based on αSMA+ expression in E0771 tumours. We found that some CAFs in these tumours express AT1 at high levels, whereas other cells express AT1 at low levels. Colocalization is shown in yellow. Scale bar, 25 μm. (g) Expression of AT2 (red) in αSMA+ CAFs (green) and cancer cells in tumours. Most CAFs express high levels of AT2, whereas some other cells express similar AT2 levels. Colocalization is shown in yellow. Scale bar, 25 μm. Animal numbersn=4–5. Error bars indicate s.e.m. Figure 4: Stromal angiotensin signalling induces matrix production in tumours. ( a ) Tumour collagen and ( b ) hyaluronan levels in angiotensin-II-receptor-1 (AT1)-knockout mice. Orthotopic E0771 breast tumours implanted in AT1-knockout mice ( Agtr1a −/− ) have ( a ) a lower collagen I area fraction (* P= 0.026, Student’s t -test) and ( b ) a lower hyaluronan area fraction (* P= 0.011, Student’s t -test) than E0771 tumours implanted in wild-type C57BL/6 mice. ( c ) Tumour collagen and ( d ) hyaluronan levels in angiotensin-II-receptor-2 (AT2) knockout mice. Orthotopic E0771 breast tumours implanted in AT2-knockout mice ( Agtr2 −/− ) have ( c ) a higher collagen I area fraction (* P= 0.047, Student’s t -test) and ( d ) a higher hyaluronan area fraction (* P= 0.012, Student’s t -test) than E0771 tumours implanted in wild-type C57BL/6 mice. Tumours were time- and size-matched at ~200 mm 3 . ( e ) Expression of AT1 ( Agtr1a and Agtr1b genes) and AT2 ( Agtr2 gene) mRNA in murine cancer-associated fibroblasts (CAFs) and cancer cells. CAFs isolated from AK4.4 tumours express over one order of magnitude more AT1 than either E0771 or AK4.4 cancer cells. Similarly, the CAFs express over two orders of magnitude more AT2 than either E0771 or AK4.4 cells. ( f ) Expression of AT1 (red) in αSMA+ CAFs (green) and cancer cells in tumours. We imaged CAFs based on αSMA+ expression in E0771 tumours. We found that some CAFs in these tumours express AT1 at high levels, whereas other cells express AT1 at low levels. Colocalization is shown in yellow. Scale bar, 25 μm. ( g ) Expression of AT2 (red) in αSMA+ CAFs (green) and cancer cells in tumours. Most CAFs express high levels of AT2, whereas some other cells express similar AT2 levels. Colocalization is shown in yellow. Scale bar, 25 μm. Animal numbers n =4–5. Error bars indicate s.e.m. Full size image Angiotensin inhibition lowers solid stress in tumours We next investigated the effects of losartan on solid stress in tumours. We measured solid stress in these tumours using our recently established technique [5] . Losartan reduced solid stress in both E0771 and AK4.4 tumours ( Fig. 5a ), as well as in 4T1 breast and Pan-02 pancreatic tumours ( Fig. 5b ). We additionally tested a panel of ARBs and found that they all reduced solid stress ( Supplementary Fig. S10 ), further suggesting that the mechanism of action is via AT1 inhibition rather than an off-target effect of losartan. These data indicate that angiotensin blockers may be capable of decompressing vessels in desmoplastic tumours by reducing solid stress through their antimatrix effects. 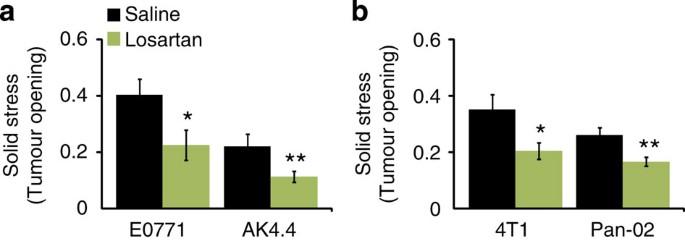Figure 5: Losartan targets solid stress in tumours. (a) Solid stress levels in tumours after angiotensin inhibition using losartan. Solid stress was assessed using anex vivotechnique involving the measurement of the extent of tumour tissue relaxation (tumour opening relative to tumour diameter) following a stress-releasing incision, with larger openings indicating higher stress5. Through its antimatrix effects, losartan reduces solid stress in E0771 (*P=0.049, Student’st-test) and AK4.4 (**P=0.043, Student’st-test). (b) Losartan reduces solid stress in additional models, including 4T1 breast tumours (*P=0.036, Student’st-test) and Pan-02 pancreatic tumours (**P=0.0092, Student’st-test). Animal numbersn=5 (E0771),n=8–9 (AK4.4),n=10–11 (4T1),n=4–8 (Pan-02). Error bars indicate s.e.m. Figure 5: Losartan targets solid stress in tumours. ( a ) Solid stress levels in tumours after angiotensin inhibition using losartan. Solid stress was assessed using an ex vivo technique involving the measurement of the extent of tumour tissue relaxation (tumour opening relative to tumour diameter) following a stress-releasing incision, with larger openings indicating higher stress [5] . Through its antimatrix effects, losartan reduces solid stress in E0771 (* P= 0.049, Student’s t -test) and AK4.4 (** P= 0.043, Student’s t -test). ( b ) Losartan reduces solid stress in additional models, including 4T1 breast tumours (* P= 0.036, Student’s t -test) and Pan-02 pancreatic tumours (** P= 0.0092, Student’s t -test). Animal numbers n =5 (E0771), n =8–9 (AK4.4), n =10–11 (4T1), n =4–8 (Pan-02). Error bars indicate s.e.m. Full size image Angiotensin inhibition decompresses tumour blood vessels We hypothesized that the reduction in solid stress by losartan would increase vascular perfusion in our desmoplastic tumour models. We found these tumours to be severely hypoperfused ( Supplementary Fig. S4 ): only 23% of vessels in E0771 breast tumours and 21% in AK4.4 pancreatic tumours were perfused with blood ( Fig. 6a,b ). Of note, collagen-rich areas seemed to colocalize with low-perfusion areas ( Fig. 3a ). Losartan significantly improved the perfused vessel fraction to 43% in E0771 and 45% in AK4.4 ( Fig. 6a,b ). Losartan treatment also increased the fraction of vessels with open lumen in E0771 and AK4.4 ( Fig. 6c ), further indicating vascular decompression as the mechanism of action [9] . Interestingly, the open lumen fraction was higher than the perfused vessel fraction in both models—perhaps because of collapse or occlusion in feeding vessels or flow cessation and clot formation [1] . Importantly, losartan did not significantly improve perfusion in the well-perfused L3.6pl tumour model, which has low collagen and 68% vessel perfusion at baseline ( Supplementary Fig. S11 ), confirming the findings of our previous study [14] . Thus, losartan can increase blood perfusion in tumours by opening existing collapsed blood vessels. 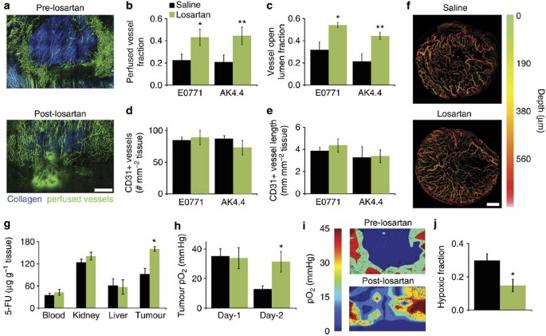Figure 6: Losartan decompresses tumour vessels to increase drug and oxygen delivery. (a) Representative images from intravital multiphoton microscopy of perfused tumour vessels (green) and collagen (blue), showing that losartan increases the density of perfused vessels in an E0771 breast tumour. Scale bar, 1 mm. (b) Perfused vessel fractions after angiotensin inhibition using losartan. Losartan increases the fraction of vessels that are perfused in orthotopic E0771 breast (*P=0.038, Student’st-test) and AK4.4 pancreatic (**P=0.039, Student’st-test) tumours. (c) Losartan also increases the fraction of vessels with open lumen in E0771 (*P=0.040, Student’st-test) and AK4.4 (**P=0.015, Student’st-test) tumours, indicating decompression as the mechanism9. (d) Vessel density and (e) vessel length following angiotensin inhibition using losartan. Losartan does not affect vessel density, as quantified by the vessel number density (d) and the total vessel length (e), indicating no antiangiogenic effect at this 40 mg kg−1dose. (f) Representative images from intravital optical frequency-domain imaging of perfused vessels with losartan treatment. E0771 tumours in control mice have a low density and poor distribution of perfused vessels in three dimensions, whereas losartan-treated mice showed a more even distribution and higher density of perfused vessels. Scale bar, 1 mm. (g) Small-molecule drug delivery to tumours and various organs after angiotensin inhibition with losartan. Losartan increases the accumulation of the small-molecule chemotherapeutic 5-FU in AK4.4 pancreatic tumours by 74% (*P=0.0063, Student’st-test), while not affecting accumulation in the normal organs. (h) Oxygen delivery to tumours measured by phosphorescence quenching microscopy during angiotensin inhibition using losartan, with (i) representative images. Losartan maintains the level of oxygenation (h) in the tissue, versus control tumours that become progressively more hypoxic with time (*P=0.030, Student’st-test) as the tumours grow from 3 to 5 mm in diameter. Losartan increases oxygenation in some tumours (i) whereas all control tumours decrease in oxygen levels. Losartan also appears to result in a more homogenous distribution of well-oxygenated tumour tissue. Scale bar, 100 μm. (j) Hypoxic fraction in tumours measured by pimonidazole injection and staining following angiotensin inhibition with losartan. Losartan decreases the hypoxic fraction in E0771 tumours (*P=0.019, Student’st-test) because of the increase in oxygen delivery. Animal numbersn=7–9 (vessels),n=4–5 (vessel lumen),n=4 (drug delivery),n=6 (oxygen delivery),n=6–7 (hypoxia). Error bars indicate s.e.m. Figure 6: Losartan decompresses tumour vessels to increase drug and oxygen delivery. ( a ) Representative images from intravital multiphoton microscopy of perfused tumour vessels (green) and collagen (blue), showing that losartan increases the density of perfused vessels in an E0771 breast tumour. Scale bar, 1 mm. ( b ) Perfused vessel fractions after angiotensin inhibition using losartan. Losartan increases the fraction of vessels that are perfused in orthotopic E0771 breast (* P= 0.038, Student’s t -test) and AK4.4 pancreatic (** P= 0.039, Student’s t -test) tumours. ( c ) Losartan also increases the fraction of vessels with open lumen in E0771 (* P= 0.040, Student’s t -test) and AK4.4 (** P= 0.015, Student’s t -test) tumours, indicating decompression as the mechanism [9] . ( d ) Vessel density and ( e ) vessel length following angiotensin inhibition using losartan. Losartan does not affect vessel density, as quantified by the vessel number density ( d ) and the total vessel length ( e ), indicating no antiangiogenic effect at this 40 mg kg −1 dose. ( f ) Representative images from intravital optical frequency-domain imaging of perfused vessels with losartan treatment. E0771 tumours in control mice have a low density and poor distribution of perfused vessels in three dimensions, whereas losartan-treated mice showed a more even distribution and higher density of perfused vessels. Scale bar, 1 mm. ( g ) Small-molecule drug delivery to tumours and various organs after angiotensin inhibition with losartan. Losartan increases the accumulation of the small-molecule chemotherapeutic 5-FU in AK4.4 pancreatic tumours by 74% (* P= 0.0063, Student’s t -test), while not affecting accumulation in the normal organs. ( h ) Oxygen delivery to tumours measured by phosphorescence quenching microscopy during angiotensin inhibition using losartan, with ( i ) representative images. Losartan maintains the level of oxygenation ( h ) in the tissue, versus control tumours that become progressively more hypoxic with time (* P= 0.030, Student’s t -test) as the tumours grow from 3 to 5 mm in diameter. Losartan increases oxygenation in some tumours ( i ) whereas all control tumours decrease in oxygen levels. Losartan also appears to result in a more homogenous distribution of well-oxygenated tumour tissue. Scale bar, 100 μm. ( j ) Hypoxic fraction in tumours measured by pimonidazole injection and staining following angiotensin inhibition with losartan. Losartan decreases the hypoxic fraction in E0771 tumours (* P= 0.019, Student’s t -test) because of the increase in oxygen delivery. Animal numbers n =7–9 (vessels), n =4–5 (vessel lumen), n =4 (drug delivery), n =6 (oxygen delivery), n =6–7 (hypoxia). Error bars indicate s.e.m. Full size image Despite the previous classification of angiotensin inhibitors as antiangiogenics [32] , we found that losartan did not reduce vascular endothelial growth factor (VEGF) levels ( Supplementary Fig. S12 ), affect the CD31+ vessel density in these tumours ( Fig. 6d,e ) or decrease vessel diameter ( Supplementary Fig. S13 ). Further, losartan increased the effective permeability of the blood vessels for all sizes of nanoparticles ( Supplementary Fig. S14 ), which is inconsistent with the ‘vascular normalization’ effect that results from antiangiogenic therapy [33] . Moreover, this dose did not decrease blood pressure in a separate group of tumour-bearing mice with advanced disease ( Supplementary Fig. S15 ) [14] , and correspondingly did not affect flow rates in individual blood vessels ( Supplementary Fig. S16 ). As such, we confirmed that losartan does not improve perfusion by reducing vessel leakiness or increasing blood flow, as seen after vascular normalization [11] , [33] , but rather does so through ‘microenvironmental normalization’. Angiotensin inhibitors enhance drug and oxygen delivery As drug and oxygen delivery to tissues is governed by vascular perfusion, we tested the effects of losartan on delivery to tumours. We first engaged a mathematical approach to analyse the efficiency of the vascular network for drug and oxygen delivery. Using multiphoton microscopy, we imaged the perfused vessel networks of E0771 tumours ( Fig. 6a ). On the basis of metrics of intervascular spaces [34] , we found that losartan reduces the distance drugs and oxygen must travel to reach tumour cells ( Fig. 6f and Supplementary Fig. S17 ). We then measured the total tissue accumulation of the small-molecule chemotherapeutic fluorouracil (5-fluorouracil; 5-FU). Losartan improved 5-FU delivery to AK4.4 tumours while not affecting delivery to normal organs ( Fig. 6g ). These data imply that this strategy for enhancing delivery selectively affects tumours, which is expected, since solid stress does not accumulate in most normal organs [5] . We then studied oxygenation using phosphorescence quenching microscopy [35] . We found that losartan treatment maintained tumour oxygen levels in E0771 tumours, whereas control-treated tumours showed a typical growth-dependent drop in oxygenation ( Fig. 6h,i ). We confirmed this decrease in tumour hypoxia by using pimonidazole staining in E0771 and 4T1 ( Fig. 6j and Supplementary Figs S18 and S19 ). Thus, reducing solid stress through ‘microenvironmental normalization’ with angiotensin inhibitors increases the delivery of drugs and oxygen to tumours. Angiotensin inhibition potentiates chemotherapy Given these effects on delivery, we tested losartan in combination with doxorubicin in E0771 and 4T1 tumours, or with 5-FU in AK4.4 tumours. We found that the combination of losartan with chemotherapy significantly delayed E0771, 4T1 and AK4.4 tumour growth, whereas monotherapy had no effect ( Fig. 7a–c and Supplementary Fig. S20 ). Moreover, the combination of losartan and chemotherapy increased median survival (time to death or excessive tumour burden) for mice bearing E0771 and 4T1 tumours compared with monotherapy ( Fig. 7d,e ). Similarly, the combination increased median survival (time to death) for mice bearing AK4.4 tumours, whereas monotherapy did not extend survival ( Fig. 7f ). Importantly, losartan alone—despite increasing blood perfusion—did not shorten survival in any model. The results of the combination for survival were somewhat better than for primary tumour growth delay, indicating a possible effect on metastases. Correspondingly, losartan slightly decreased metastasis in E0771 ( Supplementary Fig. S21 ), consistent with previous studies [36] and probably because of the role of angiotensin signalling in promoting the metastatic cascade [37] , [38] . Of note, we found that losartan combined with doxorubicin delayed tumour growth in both immunodeficient and immunocompetent models of breast cancer ( Fig. 7a,b and Supplementary Fig. S21 ), although the effects appeared less pronounced in immunocompetent mice even at high doses of doxorubicin. This might be attributed to resistance induced by the immune microenvironment [39] . Together, these data demonstrate that angiotensin inhibitors can improve the effectiveness of small-molecule chemotherapeutics through antimatrix effects. 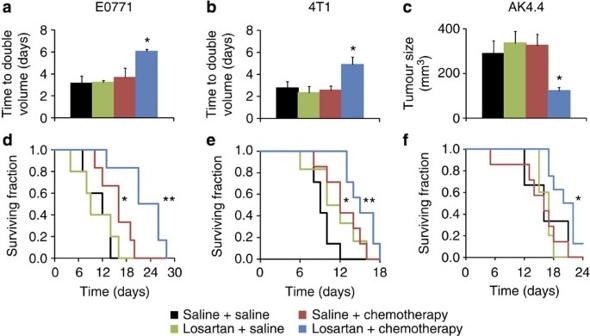Figure 7: Losartan potentiates chemotherapy. (a) Quantification of tumour growth rates, based on the time to reach double the initial volume, for orthotopic E0771 breast tumours in response to treatment with losartan or saline control (40 mg kg−1daily from day 0 onwards) in combination with either the small-molecule chemotherapeutic doxorubicin or saline control (2 mg kg−1every 3 days from day 1 onwards). Doxorubicin and losartan monotherapy induce no significant growth delay versus the control treatment in these aggressive tumours. In contrast, their combination greatly limits tumour growth (*P=0.040, Student’st-test). (b) Quantification of tumour growth rates, based on the time to reach double the initial volume, for orthotopic 4T1 breast tumours using the same treatments as with E0771. Doxorubicin and losartan monotherapy induce no significant growth delay versus the control treatment. In contrast, their combination greatly limits tumour growth (*P=0.024, Student’st-test). (c) Volumes of orthotopic AK4.4 pancreatic tumours on day 7 in response to treatment with losartan or saline control (40 mg kg−1daily from day 0 to 7) in combination with either the small-molecule chemotherapeutic 5-FU or saline control (60 mg kg−1on days 2 and 6). 5-FU and losartan monotherapy induce no significant growth delay versus the control treatment, whereas their combination greatly inhibited tumour growth (*P=0.0085, Student’st-test). (d) Animal survival for E0771-bearing mice following the initiation of treatment. Doxorubicin monotherapy improves survival versus the control (*P=0.048, log-rank test), whereas the combination of doxorubicin and losartan enhances this survival increase versus doxorubicin monotherapy (**P=0.014, log-rank test). (e) Animal survival for 4T1-bearing mice following the initiation of treatment. Doxorubicin monotherapy improves survival versus the control (*P=0.045, log-rank test), whereas the combination of doxorubicin and losartan enhances this survival increase versus doxorubicin monotherapy (**P=0.050, log-rank test). (f) Animal survival for AK4.4-bearing mice following the initiation of treatment. The combination of 5-FU and losartan enhances survival versus 5-FU (*P=0.019, log-rank test) or losartan monotherapy (*P=0.027, log-rank test). Animal numbersn=5–6 (E0771, AK4.4 growth),n=3–8 (AK4.4 survival),n=6–7 (4T1). Error bars indicate s.e.m. Statistical tests were corrected for multiple comparisons using the Holm–Bonferroni method. Figure 7: Losartan potentiates chemotherapy. ( a ) Quantification of tumour growth rates, based on the time to reach double the initial volume, for orthotopic E0771 breast tumours in response to treatment with losartan or saline control (40 mg kg −1 daily from day 0 onwards) in combination with either the small-molecule chemotherapeutic doxorubicin or saline control (2 mg kg −1 every 3 days from day 1 onwards). Doxorubicin and losartan monotherapy induce no significant growth delay versus the control treatment in these aggressive tumours. In contrast, their combination greatly limits tumour growth (* P= 0.040, Student’s t -test). ( b ) Quantification of tumour growth rates, based on the time to reach double the initial volume, for orthotopic 4T1 breast tumours using the same treatments as with E0771. Doxorubicin and losartan monotherapy induce no significant growth delay versus the control treatment. In contrast, their combination greatly limits tumour growth (* P= 0.024, Student’s t -test). ( c ) Volumes of orthotopic AK4.4 pancreatic tumours on day 7 in response to treatment with losartan or saline control (40 mg kg −1 daily from day 0 to 7) in combination with either the small-molecule chemotherapeutic 5-FU or saline control (60 mg kg −1 on days 2 and 6). 5-FU and losartan monotherapy induce no significant growth delay versus the control treatment, whereas their combination greatly inhibited tumour growth (* P= 0.0085, Student’s t -test). ( d ) Animal survival for E0771-bearing mice following the initiation of treatment. Doxorubicin monotherapy improves survival versus the control (* P =0.048, log-rank test), whereas the combination of doxorubicin and losartan enhances this survival increase versus doxorubicin monotherapy (** P =0.014, log-rank test). ( e ) Animal survival for 4T1-bearing mice following the initiation of treatment. Doxorubicin monotherapy improves survival versus the control (* P =0.045, log-rank test), whereas the combination of doxorubicin and losartan enhances this survival increase versus doxorubicin monotherapy (** P =0.050, log-rank test). ( f ) Animal survival for AK4.4-bearing mice following the initiation of treatment. The combination of 5-FU and losartan enhances survival versus 5-FU (* P =0.019, log-rank test) or losartan monotherapy (* P =0.027, log-rank test). Animal numbers n =5–6 (E0771, AK4.4 growth), n =3–8 (AK4.4 survival), n =6–7 (4T1). Error bars indicate s.e.m. Statistical tests were corrected for multiple comparisons using the Holm–Bonferroni method. Full size image This study highlights the complex role of the tumour matrix as a drug delivery barrier. Although the distribution of larger drugs such as nanomedicines is hindered by steric interactions with collagen, the matrix does not directly limit the distribution of smaller, conventional chemotherapeutics [40] . Rather, the matrix indirectly limits the delivery of conventional chemotherapy through vascular compression. Both hyaluronan and collagen fibres contribute to solid stress in tumours: hyaluronan does so by resisting compression, whereas collagen does so by resisting tension and confining the local microenvironment [5] . Our results lead to a new model for how hyaluronan and collagen affect vessel compression. As cancer and stromal cells proliferate, they attempt to expand their local tumour microenvironment, exerting tensile stress. This tensile stress stretches collagen fibres in the microenvironment, which store tensile elastic ‘strain’ energy and stiffen, thereby resisting this expansion. The effect is to confine these cells such that the force they generate while proliferating becomes a compressive stress. These cells cannot transmit compressive stress perpendicularly to the fibres of this stiffened collagen; hence, this compressive stress is instead exerted largely on hyaluronan in the local tumour microenvironment. Hyaluronan, whose internal charges repel each other electrostatically and trap water molecules, resists this compression, only storing compressive ‘strain’ energy until maximally compressed. Beyond this maximal compression, the excess compressive stress is transmitted by hyaluronan to tumour vessels. These tumour vessels, which lack the complete coverage by pericytes and basement membrane that fortifies mature vessels, are structurally weak and cannot resist compression. If collagen levels are low in a tumour, the microenvironment is more easily expanded by proliferating cells and thus compressive stress is not produced to as high a level. As a result, hyaluronan does not contribute to vessel compression in collagen-poor tumours. If hyaluronan levels are low, the compressive stress is not transmitted to vessels to as great a degree. Thus, hyaluronan seems responsible for transmitting compressive stress to vessels in all cases when there is no direct cell contact, whereas collagen enables compressive stress to be applied to hyaluronan by cells. Analyses of retrospective clinical data suggest that the use of AT1 blockers (ARBs) and ACE-Is to manage hypertension in cancer patients receiving standard therapies is correlated with longer survival in pancreatic and other cancers [41] , [42] , [43] , as well as a reduced risk of recurrence in breast cancer [44] . However, a causal relationship between the use of ARBs/ACE-Is and its clinical benefit—as well as the mechanism behind this potential effect—has not been revealed. AT1 signalling has been shown to increase VEGF expression by CAFs [45] , and both ACE-Is and ARBs can decrease VEGF expression and angiogenesis [46] , [47] . It has therefore been assumed that their indirect antiangiogenic properties, through downstream VEGF inhibition, benefit survival additively. Our current findings, in line with our previous report [14] , do not support this antiangiogenic mechanism. Further, we detected no growth delay or survival benefit with losartan monotherapy in our study. This is in contrast to the ability of angiotensin signalling through AT1 to promote tumour growth and metastasis [32] , [37] , [38] , [48] , [49] , with signalling through AT2 hindering growth [50] . This is perhaps because these growth inhibitory effects are primarily seen at much higher doses of ARBs [36] , [46] , [51] or with long-term treatment [52] ; indeed, when used at low doses, ARBs have been shown by others to not cause a growth delay [47] . It is also possible that this VEGF inhibition is because of direct effects of angiotensin inhibitors on cancer cells, and that our models do not respond similarly because the cancer cells used do not express high levels of AT1 or AT2. These inconsistent data notwithstanding, it should be noted that antiangiogenic therapy with bevacizumab has failed to prolong survival in desmoplastic tumours such as breast and pancreatic cancer [3] , casting doubt on a possible antiangiogenic mechanism for the benefits observed with angiotensin inhibitors. Here we have found that angiotensin inhibitors actually increase vessel perfusion through vascular decompression, doing so by reducing stromal activity and production of matrix components responsible for compression. Notably, these drugs are the first to target all stromal components (CAFs, hyaluronan and collagen) known to contribute to solid stress [5] . Our findings also suggest that AT2 agonists or inhibitors of downstream signalling through TGF-β1, CCN2 or ET-1 may similarly reduce solid stress to enhance chemotherapy, although such agents have not been tested in this way. Similarly, angiotensin (1–7), a MAS agonist that can reduce CAF matrix production, may be useful for targeting solid stress [53] . Meanwhile, there are challenges to address for translation. Deleterious effects on blood pressure may contraindicate angiotensin inhibitors for some patients [14] , [54] . Further, we expect that angiotensin inhibitor distribution into tumours may be the most important factor controlling efficacy: drugs displaying a lack of tissue penetration (such as candesartan) would therefore be poor candidates relative to those with high penetration (such as losartan and telmisartan) [55] . Indeed, the inadequate tumour penetration of candesartan may explain why it only improved chemotherapy outcomes modestly, when comparing high versus low candesartan doses, in a recent pancreatic cancer study [54] . These factors are why losartan was selected over other angiotensin inhibitors for a recently initiated clinical trial in pancreatic cancer (NCT01821729) at Massachusetts General Hospital. Regardless, the safety and low cost of ARBs and ACE-Is—along with their potentiation of conventional chemotherapy—make a strong case for repurposing angiotensin inhibitors as adjuncts for cancer therapies. Drug preparation Angiotensin inhibitors (losartan, lisinopril, valsartan and candesartan) were obtained as pills, crushed and dissolved in PBS (for losartan and lisinopril) or PBS with 5% ethanol (for valsartan and candesartan) over 24 h. The solutions were then sterile filtered for injection. Doxorubicin and 5-FU were obtained as solutions for injection. All drugs were purchased from the pharmacy at Massachusetts General Hospital. Tumour models AK4.4 cells ( Kras G12D and p53 +/− ) were kindly provided by Dr Nabeel Bardeesy, and were isolated from mice generating spontaneous pancreatic tumours [56] ( Ptf1-Cre/LSL-Kras G12D /p53 Lox/+ ). Orthotopic pancreatic tumours were generated by implanting a small piece (1 mm 3 ) of viable tumour tissue (from a source tumour in a separate animal) into the pancreas of a 6–8-week-old male FVB (AK4.4 model) or C57BL/6 (Pan-02 model) mouse. Orthotopic breast tumours were similarly generated by implanting a chunk of viable tumour tissue into the mammary fat pad of a 6–8-week-old female severe combined immunodeficient (SCID) mouse (E0771 and 4T1 models) or C57BL/6 mouse (E0771 syngeneic model). For AT1- and AT2-knockout studies, E0771 cells were implanted by injection into the mammary fat pad of 6–8-week-old female C57BL/6, agtr1a −/− (ref. 57 ) or agtr2 −/− (ref. 58 ) mice. All animal procedures were carried out following the Public Health Service Policy on Humane Care of Laboratory Animals and approved by the Institutional Animal Care and Use Committee of Massachusetts General Hospital. Vessel perfusion and hypoxia histology For breast tumours, mice bearing orthotopic E0771 were split into time- and size-matched (~100 mm 3 ) treatment groups. For pancreatic tumours, mice bearing orthotopic AK4.4 were split into treatment groups 6 days post implantation. The mice were then treated with 40 mg kg −1 losartan or an equal volume of PBS intraperitoneally each day for 6 (E0771) or 7 (AK4.4) days. On the day of the last treatment, mice were slowly (~2 min) injected with 100 μl of 1 mg ml −1 biotinylated lectin (Vector Labs), administered via the retro-orbital sinus 5 min before tumour removal. For hypoxia studies, the mice were also injected with 60 mg kg −1 of pimonidazole at 10 mg ml −1 1 h before tumour removal. The tumours were then excised, fixed in 4% formaldehyde in PBS (30 min mm −1 diameter of tissue), incubated in 30% sucrose in PBS overnight at 4 °C and frozen in optimal cutting temperature compound (Tissue-Tek). Transverse tumour sections, 40 μm thick, were immunostained with antibodies to endothelial marker CD31 (MEC13.3 antibody, Biosciences (BD), 1:100 dilution) and counterstained with 4',6-diamidino-2-phenylindole (Vector Labs). Collagen I and hyaluronan were, respectively, detected using the LF-68 antibody (1:50 dilution) provided by Dr Larry Fisher (NIDCR) and a biotinylated hyaluronan proteoglycan fragment (385911, Calbiochem), as previously described [40] . Staining for αSMA (C6198 antibody, Sigma, 1:100 dilution), active TGF-β1 (G122A antibody, Promega, 1:15 dilution), CCN2 (TP-243 antibody, Torrey Pines, 1:100 dilution), AT1 (ab18801 antibody, Abcam, 1:100 dilution) and AT2 (AAR-012 antibody, Alomone, 1:200 dilution) were carried out in 10 μm sections. For the detection of collagen I in AK4.4, KPC and human pancreatic ductal adenocarcinoma, the paraffin-embedded sections were treated with a pH-9.0 antigen retrieval solution and counterstained with haematoxylin. Histological image analysis Eight random fields (four interior and four periphery) at × 20 magnification were taken from each slide using a confocal microscope (Olympus). For vascular analysis, vessels were skeletonized and segmented using a custom, semi-automated tracing program developed in MATLAB (The MathWorks), allowing the removal of structures under 30 pixels and regions of autofluorescence. For perfusion fraction, the number of vessels counted by this program with colocalization of lectin and CD31 staining was divided by the number of vessels counted with CD31 staining. For vessel metrics, including diameter and density, the program determined the average size of all counted vessels and their length, as well as the count per area. For open versus closed lumen quantification, vessels were analysed by eye and a vessel was counted as open if it had a clearly visible lumen throughout its length. Images of collagen I, hyaluronan, pimonidazole (hypoxia) αSMA, active-TGF-β1 and CCN2-stained sections were analysed based on the area fraction of positive staining. Identical analysis settings and thresholds were used for all tumours. CAF studies We generated αSMA P -dsRed/Tie2 P -GFP/ FVB double-transgenic mice by crossing Tie2 P -GFP/ FVB mice [59] with αSMA P -dsRed mice [19] . Once established, this line was backcrossed to FVB mice for at least 10 generations. CAFs were isolated from AK4.4 tumours implanted in 6–8-week-old male mice of this line. The mice were treated with 40 mg kg −1 losartan or PBS for 7 days, and then the tumours were collected and αSMA+ cells were isolated based on dsRed fluorescence using fluorescence-activated cell sorting (BD Biosciences). These cells were analysed with quantitative reverse transcriptase-PCR for messenger RNA of Col1a1 (F 5′-GCTCCTCTTAGGGGCCACT-3′, R 5′-CCACGTCTCACCATTGGGG-3′), Has1 (F, 5′-GGCGAGCACTCACGATCATC-3′, R 5′-AGGAGTCCATAGCGATCTGAAG-3′), Has2 (F 5′-TGTGAGAGGTTTCTATGTGTCCT-3′, R 5′-ACC GTA CAG TCC AAA TGA GAA GT-3′), Has3 (F 5′-CCTGGAGCACCGTCGAATG-3′, R 5′-CCTTGAGGTTTGGAAAGGCAA-3′), Tgfb1 (F 5′-GCAGTGGCTGAACCAAGGA-3′, R 5′-AGCAGTGAGCGCTGAATCG-3′), Ctgf (F 5′-CAAAGCAGCTGCAAATACCA-3′, R 5′-GTCTGGGCCAAATGTGTCTT-3′) and Edn1 (F 5′-GCACCGGAGCTGAGAATGG-3′, R 5′-GTGGCAGAAGTAGACACACTC-3′). We also analysed these cells, as well as AK4.4 and E0771 cells, for Agtr1a (F 5′-AACAGCTTGGTGGTGATCGTC-3′, R 5′-CATAGCGGTATAGACAGCCCA-3′), Agtr1b (F 5′-TGGCTTGGCTAGTTTGCCG-3′, R 5′-ACCCAGTCCAATGGGGAGT-3′) and Agtr2 (F 5′-AACTGGCACCAATGAGTCCG-3′, R 5′-CCAAAAGGAGTAAGTCAGCCAAG-3′). Expression levels were normalized to the control (GAPDH) and losartan-treated levels were normalized to the PBS controls. Solid stress Solid stress was measured using the tumour opening technique [5] . When the tumours reached a size of ~1 cm in diameter, the mice were anaesthetized. Subsequently, each tumour was excised, washed with Hank’s balanced salt solution and its three dimensions were measured. Each tumour was cut along its longest axis, to a depth of 80% of its shortest dimension, using a scalpel. The tumours were allowed to relax for 10 min in Hank’s balanced salt solution to diminish any transient, poro-elastic responses. Afterwards, the opening resulting from the cut was measured at the middle of the cut at the surface of the tumour. Solid stress is proportional to the size of the opening relative to the size of the dimension perpendicular to the cut. Drug delivery Mice bearing orthotopic AK4.4 were split into treatment groups 6 days after implantation. The mice were then treated with 40 mg kg −1 losartan or an equal volume of PBS intraperitoneally each day for 7 days. On the day of the last treatment, mice were injected with 100 mg kg −1 5-FU, administered retro-orbitally 30 min before tumour and organ removal. The tissue was dabbed of excess blood and then snap-frozen in liquid nitrogen for analysis. 5-FU was isolated from the tissues and measured using liquid–liquid extraction followed by reverse-phase HPLC with tandem mass-spectrometry. In vivo imaging For imaging studies, E0771 tumours were implanted in mice bearing mammary fat pad chambers [33] and allowed to grow to ~3 mm in diameter. Multiphoton imaging was carried out on a custom-built multiphoton laser-scanning microscope using a confocal laser-scanning microscope body (Olympus 300, Optical Analysis) and a broadband femtosecond laser source (High Performance MaiTai, Spectra-Physics) [60] . Images were taken at ~60 mW at sample surface. Mosaic images were taken in raster pattern using a motorized stage (H101, Prior Scientific, Inc.) and customized automation software (LabView, National Instruments). Imaging studies were performed with a × 20 magnification, 0.95 NA water immersion objective (Olympus XLUMPlanFl, 1-UB965, Optical Analysis). Optical frequency-domain imaging was carried out after 7 days of treatments using a custom-built microscope [61] . Tissue oxygenation We measured pO2 in the tumours using phosphorescence quenching microscopy [35] , which was adapted to multiphoton microscopy. An oxygen-sensitive porphyrin, Oxyphor R2 (Oxygen Enterprises) was injected retro-orbitally 12 h before imaging, and was reinjected immediately before imaging along with 2 MDa fluorescein isothiocyanate-dextran (Sigma-Aldrich) for functional vascular tracing. A mosaic image of the tumour was collected, and oxygen was then measured in an evenly spaced 12 × 12 grid at four depths (60, 120, 180 and 240 μm) in the tumour. At each point in the grid, the phosphorescence lifetime of the probe was measured after each of several repeated brief intense pulses of 1,020 nm laser light, and these lifetime measurements were combined. A two-component model was used to calculate the oxygen tension from each lifetime measurement, accounting for binding and quenching of the probe by both oxygen and proteins. The grid was then overlaid on the mosaic to make an oxygen map. Effective permeability Effective permeability (transvascular flux) studies were carried out using a mixture of nanoparticles with diameters of 12 nm (476 nm emission), 60 nm (540 nm emission) and 125 nm (625 nm emission) [33] . Concentrations were adjusted with in vitro calibration to result in roughly equal photoluminescence intensity for all three nanoparticle samples under 800 nm multiphoton excitation. Following retro-orbital injection of 200 μl with these concentrations, multiphoton imaging was carried out as described above at depths from 0 to 201 μm, with 2.76 μm steps and 2.76 × 2.76 μm pixels. Images were taken every 3 min at each region of interest for a duration of 1 h. Images were analysed using custom analysis software developed in Matlab (The MathWorks) [33] , [62] . The analysis approach involved three-dimensional (3D) vessel tracing to create vessel metrics and a 3D map of voxel intensity versus distance to the nearest vessel over time. Images were also corrected for sample movement over time with 3D image registration. The effective permeability (normalized transvascular flux) was calculated using , where J t is the transvascular flux, S v is the vessel surface area, C v is the concentration of the probe in the vessel, C is the concentration of the probe immediately extravascular, P eff is the effective permeability, t is the time after the initial image, r is the distance from the vessel central axis and R is the vessel radius at that point along the vessel. Fluorescence intensities were used as these concentrations. The calculation was made as an average over the entire imaged volume for each tumour. Individual tumour vessel blood flow Red blood cell (RBC) velocity was measured using intravital microscopy with the residence time line scanning technique in mice bearing orthotopic E0771 or 4T1 mammary tumours [63] . RBCs from a donor mouse were labelled ex vivo with 1,1'-dioctadecyl-3,3,3',3'-tetramethylindodicarbocyanine perchlorate. These labelled RBCs were administered to mice bearing orthotopic E0771 or 4T1 mammary tumours via retro-orbital injection at a ratio of 3–5 labelled RBCs per 100 RBCs. Multiphoton imaging was carried out, applying laser scanning along a single line that intersects each vessel of interest. Repeated scanning along this line generated fluorescence intensity data along the line over time ( x – t ), in which ‘images’ of the fluorescent RBCs are compressed or elongated depending on the residence time of the cells in the scan. Velocities were extracted using , where v rbc is the RBC velocity, L rbc is the RBC length (7 μm), f is the line scan frequency (scans s −1 ), n scans is the number of consecutive scan lines that detected the RBC and α is the angle between vessel and line scan. Breast tumour growth and survival studies Mice bearing orthotopic E0771 or 4T1 breast tumours were split into treatment groups, time-matched for time after implantation and size-matched for tumour volume at this time (105 mm 3 in E0771 and 141 mm 3 in 4T1). The mice were then treated with 40 mg kg −1 losartan or an equal volume of PBS intraperitoneally on day 0 and each subsequent day. The mice were then treated with either 2 mg kg −1 (SCID) or 5 mg kg −1 (C57BL/6) doxorubicin, or an equal volume of saline, by intraperitonteal injection every 3 days beginning on day 1 (after two losartan or PBS treatments). Doxorubicin or control treatments were carried out 4 h after losartan or control treatments. The primary tumours were then measured every 1–2 days, beginning on day 0, using calipers. Tumour growth was quantified using the time for each to reach double (SCID) or triple (C57BL/6) its initial volume. Animal survival was quantified based on the time of death after initiation of treatment or time to reach excessive tumour burden (1000, mm 3 ). For metastasis studies, mouse lungs were collected at the killing and were fixed in Bouin’s solution. Macrometastases were counted using a stereomicroscope. Pancreatic tumour growth and survival studies Mice bearing orthotopic AK4.4 pancreatic tumours were split into treatment groups, size-matched for tumour volume (22 mm 3 ) by surgical exposure, 6 days after implantation. The mice were treated with 40 mg kg −1 losartan or an equal volume of PBS intraperitoneally on day 7 after implantation and each subsequent day. The mice were then treated with either 60 mg kg −1 5-FU or an equal volume of saline by intravenous injection on days 9 and 13 after implantation. Tumours were extracted on day 14 for measurement using calipers. Tumour growth was quantified using the size at day 14. For survival studies, mice were treated daily with losartan or PBS starting on day 3 after implantation until day 13, and then with 5-FU or saline on days 5, 9 and 13. Mean arterial pressure Mice bearing orthotopic AK4.4 pancreatic tumours were used for blood pressure measurements. Mean arterial pressure was measured by cannulation of the left carotid artery after a longitudinal skin incision above the trachea [14] . After removal of the submandibular gland, the paratracheal muscles were split and the left carotid artery was isolated. The cranial end of the artery was ligated with a 6–0 silk suture and another suture was tied loosely around the central part of the artery. A metal clamp was then positioned caudally to stop blood flow during the cannulation. A polyethylene catheter (PE-10, Becton-Dickinson) filled with heparinized saline was then inserted through a hole cut proximally to the cranial ligature, and the other suture was tied tightly around the tubing and artery. The clamp was then removed and the end of the tubing was connected to a pressure transducer for the measurement of blood pressure. Mathematical analysis and modelling The analysis was carried out on mosaic images of whole tumours taken with multiphoton microscopy after injection of 2 MDa fluorescein isothiocyanate-dextran as a perfused vessel tracer. Details of the models and corresponding equations are described in Baish et al [34] . Statistical analysis The data are presented as means with s.e. Groups were compared using a Student’s t -test, paired or unpaired, except for animal survival studies where a log-rank test was used. In pairwise comparisons within studies where multiple comparisons were made, P -values were adjusted using Holm’s method. How to cite this article: Chauhan, V.P. et al . Angiotensin inhibition enhances drug delivery and potentiates chemotherapy by decompressing tumour blood vessels. Nat. Commun. 4:2516 doi: 10.1038/ncomms3516 (2013).